Giant spin Hall effect in graphene grown by chemical vapour deposition Advances in large-area graphene synthesis via chemical vapour deposition on metals like copper were instrumental in the demonstration of graphene-based novel, wafer-scale electronic circuits and proof-of-concept applications such as flexible touch panels. Here, we show that graphene grown by chemical vapour deposition on copper is equally promising for spintronics applications. In contrast to natural graphene, our experiments demonstrate that chemically synthesized graphene has a strong spin–orbit coupling as high as 20 meV giving rise to a giant spin Hall effect. The exceptionally large spin Hall angle ~0.2 provides an important step towards graphene-based spintronics devices within existing complementary metal-oxide-semiconductor technology. Our microscopic model shows that unavoidable residual copper adatom clusters act as local spin–orbit scatterers and, in the resonant scattering limit, induce transverse spin currents with enhanced skew-scattering contribution. Our findings are confirmed independently by introducing metallic adatoms-copper, silver and gold on exfoliated graphene samples. Spintronics has been successful in the development of magnetic recording and high density magnetic memory devices [1] , [2] . The next frontier of exploration in this field is the demonstration of gate tunable control of spin currents for spin-based transistor and spin transfer torque based memory applications [3] . Key to the realization of such devices are materials with long spin relaxation times and gate tunability [4] . Graphene is an ideal material, if methods, which do not require chemical functionalization, to enhance its weak spin–orbit coupling (SOC) are devised [5] . The recent predictions of proximity enhanced SOC in graphene decorated with metallic adatoms, where electrons tunnel from graphene to adatoms and back, thereby locally enhancing the SOC, open up a new path [6] , [7] , [8] , [9] , [10] . The proximity-induced SOC in graphene decorated with physisorbed metallic adatoms is unique and different from hydrogenated graphene. In the latter case, the lattice deformation due to sp 3 hybridization results in the enhancement of SOC by Rashba [11] and sub-lattice inversion asymmetric [12] spin–orbit interactions. On the other hand, physisorbed metallic adatoms preserve the sp 2 bond character of graphene and mediate diverse spin–orbit interactions through electron tunnelling onto and off the adatoms [13] , including z →− z symmetric (intrinsic-type) and z →− z asymmetric (Rasbha-type) SOC [6] , [13] . Adatom proximity-induced SOC over the nanometre scale avoids inter-valley scattering and offers a realistic route towards two-dimensional (2D) topological insulator (TI) state engineering in graphene. The realization of such a quantum spin Hall/TI state in conjunction with the electric field effect in graphene is of great significance since TIs proximity coupled to superconductors are predicted to host Majorana fermions—an essential step towards topological quantum computations [6] . Most importantly, the detection of spin-polarized currents on the surface of TIs is a formidable task that requires the experiment to be performed in the ballistic transport regime [14] , [15] . Hence, systems with large electron mean free path in the ballistic transport regime are required. Graphene, with its ultra-high mobility even at room temperature [16] , is thus an ideal candidate for the direct experimental detection of spin-polarized currents at elevated temperatures, which until now has only been observed in 2D HgTe quantum wells at low temperatures [14] . In the following, we show that the presence of dilute residual copper (Cu) adatoms on graphene grown by chemical vapour deposition (CVD) on Cu foil (CVDG) [17] , [18] , [19] , [20] , [21] is sufficient to enhance the SOC strength by several orders of magnitude. Our experimental findings—based on Raman spectroscopy measurements, X-ray photoelectron spectroscopy (XPS), energy-dispersive X-ray spectroscopy (EDX) and non-local spin transport characterization of the samples—together with theoretical modelling demonstrate that physisorbed metallic adatoms form nanometre-size clusters [22] inducing SOC enhancement in graphene up to 20 meV. The large enhancement in SOC allows the generation of spin currents via the spin Hall effect (SHE) [23] , [24] with an exceptionally large spin Hall coefficient (angle) γ ~0.2. The latter is comparable to what has been observed in gold (Au) [25] , platinum (Pt) [26] or tungsten (W) [3] thin films with thickness at least 10 times larger than that of graphene. Here, what differentiates graphene is the strong Fermi-energy dependence of the density of states and its sharp sensitiveness to adsorbed species making it a test bed for extrinsically generated SHE [8] . To rule out CVD-specific vacancies, defects and ripples for the observed enhancement in SOC, we performed identical measurements on exfoliated pristine graphene (EPG) samples that are intentionally decorated with adatoms like copper (Cu), gold (Au) and silver (Ag; see Methods for sample preparation details). In both CVDG and EPG samples decorated with metallic adatoms, we see a similar enhancement of the SOC [27] by three orders of magnitude (up to 20 meV) confirming the proximity effect as the dominant cause for the observed SHE. 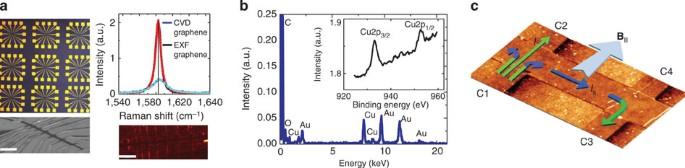Figure 1: Device characterization. (a) Optical image of 3 × 3 array of devices on Si/SiO2substrate together with the Raman and SEM image of the active area of a typical spin Hall device. Scale bar, 5 μm. (b) EDX spectrum of CVDG. The samples for EDX measurements are prepared on a standard transmission electron microscopy (TEM) gold grids and are hence suspended graphene samples. The size of each grid is 7 × 7 μm. The additional Au peaks in the EDX spectrum is due to the presence of Au TEM grids on which the graphene samples are prepared for analysis. Inset: XPS data on a CVD graphene sample showing the Cu 2p peaks. (c) AFM three-dimensional surface topography of a typical spin Hall device with details of actual measurement configurations. Device characterization Figure 1a shows the optical picture of a 3 × 3 array of CVDG spin Hall devices on a Si/SiO 2 wafer together with the Raman and scanning electron micrograph (SEM) images (see Supplementary Fig. 1 for detailed Raman mapping of the CVD samples), while Fig. 1b shows the XPS and EDX spectra for the CVDG samples. The devices consists of Hall bar arrays, such that before any spin transport measurements the CVDG devices can be first characterized for charge transport using the local four-terminal geometry with Au/Cr contacts (see Supplementary Fig. 2 and Supplementary Note 1 for details). This is followed by non-local spin transport measurements via the conventional spin-valve devices prepared in an identical manner, but using ferromagnetic electrodes [28] , [29] , [30] and MgO tunnel barriers. Such spin-valve measurements allow the independent extraction of relevant spin parameters like the spin relaxation length ( λ s ) and spin relaxation time ( τ s ) of CVDG (see Supplementary Fig. 3 and Supplementary Note 2 for details). Finally, we perform the ferromagnet free spin Hall measurements employing only Au/Cr contacts in the H-bar geometry [5] , [31] , [32] both at room temperature (RT) and at liquid-He temperatures. Figure 1: Device characterization. ( a ) Optical image of 3 × 3 array of devices on Si/SiO 2 substrate together with the Raman and SEM image of the active area of a typical spin Hall device. Scale bar, 5 μm. ( b ) EDX spectrum of CVDG. The samples for EDX measurements are prepared on a standard transmission electron microscopy (TEM) gold grids and are hence suspended graphene samples. The size of each grid is 7 × 7 μm. The additional Au peaks in the EDX spectrum is due to the presence of Au TEM grids on which the graphene samples are prepared for analysis. Inset: XPS data on a CVD graphene sample showing the Cu 2p peaks. ( c ) AFM three-dimensional surface topography of a typical spin Hall device with details of actual measurement configurations. Full size image In the H-bar geometry, a charge current ( I ) is driven across the contacts C1/C2 and a non-local voltage ( V ) is recorded across contacts C3/C4 (see Fig. 1c ). In the presence of a strong spin–orbit coupled potential V so (r), the scattering cross section σ ( θ ) for electrons with up (↑) and down (↓) spins is asymmetric, that is, σ ↑(↓) ( θ )≠ σ ↑(↓) (− θ ). This in combination with time-reversal symmetry, σ ↑(↓) ( θ )= σ ↓(↑) (− θ ), spatially separates the spin components of charge carriers leading to the formation of transverse spin current ( I s ) [8] , [33] . For a narrow channel, such that the spin relaxation length λ s is larger than the width w of the channel (λ s > w) , I s is nearly constant across w and decays along the length L as [31] where σ xx is the charge conductivity and the spin Hall conductivity. As the spins diffuse away from the source, a transverse charge accumulation is in turn induced by the inverse SHE [31] Here, is the spin Hall coefficient (angle) and is the resistivity of the sample. Hanle precession measurements, where the non-local signal is recorded as a function of an in-plane magnetic field B || are also used to unambiguously confirm that the non-local signal is indeed due to spins [31] . A minimum of five samples was measured for each type of adatoms discussed in this manuscript. Gate voltage dependence of non-local signal In Fig. 2a , we compare the non-local signals ( R NL ) as a function of the charge carrier density n at RT, for EPG and CVDG with identical length to width ratio L/w =2 and comparable mobilities (~5,000 cm 2 V −1 s −1 ). We observe an exceptionally high R NL ~160 Ω for CVDG. On the other hand, in exfoliated graphene, the measured signal is indistinguishable from the expected Ohmic contribution (~20 Ω). 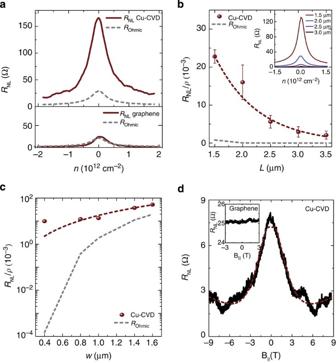Figure 2: Non-local measurements on CVD graphene. (a)RNLversusnfor pristine graphene sample (lower panel) and Cu-CVD graphene (upper panel).L/w=2 for both the samples. The grey dotted lines represent the Ohmic contribution to the non-local signals. (b)RNL/ρversusLfor CVD graphene with the widthw=500 nm. The data are mean values for three samples and the error bar corresponds to the s.d. from the mean value. Inset:RNLfor differentL/wratio of the channel. (c)RNL/ρversuswfor Cu-CVD graphene. Here,L=2 μm for all devices. The grey dotted line shows the Ohmic contribution and (d) the in-plane magnetic field dependence of the non-local signal for Cu-CVD graphene samples. The dotted line is the fit for the data using equation (6). Inset: magnetic field dependence of pristine exfoliated graphene sample. The latter follows Figure 2: Non-local measurements on CVD graphene. ( a ) R NL versus n for pristine graphene sample (lower panel) and Cu-CVD graphene (upper panel). L/w =2 for both the samples. The grey dotted lines represent the Ohmic contribution to the non-local signals. ( b ) R NL /ρ versus L for CVD graphene with the width w =500 nm. The data are mean values for three samples and the error bar corresponds to the s.d. from the mean value. Inset: R NL for different L/w ratio of the channel. ( c ) R NL / ρ versus w for Cu-CVD graphene. Here, L =2 μm for all devices. The grey dotted line shows the Ohmic contribution and ( d ) the in-plane magnetic field dependence of the non-local signal for Cu-CVD graphene samples. The dotted line is the fit for the data using equation (6). Inset: magnetic field dependence of pristine exfoliated graphene sample. Full size image where ρ is the resistivity of the device [31] , [32] . Thermo-magneto electric effects, as discussed in ref. 34 , are only present in an externally applied perpendicular magnetic field (see Supplementary Fig. 4 and Supplementary Note 3 for details). Thus, we are left with only the SHE that can give rise to such a large non-local signal at zero magnetic fields. This, however, requires a significant SOC strength and hence points to a strongly enhanced SOC in CVDG when compared with EPG. Length, width and in-plane magnetic field dependence of R NL To demonstrate the spin nature of the measured non-local signal, we next study the dependence of R NL on the device geometry. The dependence of the non-local signal on the device geometry (length and width) can be obtained by solving the diffusion equation for the spins and is given by [31] , [35] , [36] Here, λ s is the spin relaxation length and is related to the spin precession length λ so , defined as the length scale for a complete spin precession cycle in a clean system, by . The dimensional dependence of R NL , thus, allows two independent experiments: (1) the length and (2) the width dependence of the non-local signal, to extract the critical spin parameters like the spin relaxation length ( λ s ) and spin Hall angle ( γ ). In the first case, for a constant width w, equation (4) gives a R NL which decays exponentially with the length L. In the second case, where the width of the sample is varied, we chose devices with narrow width such that the condition λ s , λ so > w is satisfied. In this case, equation (4) for R NL , can be simplified by expanding the exponential term as that is, the non-local signal R NL has a power law dependence on w . Here, we first discuss the length dependence of R NL ( Fig. 2b ) by fixing w =500 nm and varying length L =1.5−4 μm. As expected, the non-local signal decays exponentially with L and the fit with equation (4) gives a λ s ~0.8 μm and a γ ~0.2. We next study the width dependence of R NL by fixing L =2 μm. Figure 2c shows R NL versus w for a device with L =2 μm at the CNP and at RT (see Supplementary Fig. 5 and Supplementary Note 4 for additional data). The observed power law behaviour in our devices again confirms the spin nature of the R NL. Noteworthy, the difference between Ohmic and measured non-local signals is more distinct in junctions with smaller width, in agreement with predictions for narrow channels, that is, λ s , λ so > w (refs 31 , 35 ). Furthermore, the values for λ s ( w (600 nm)=2 μm) and γ (0.18), obtained from the width dependence, are in good agreement with values extracted from the length dependence. For a final and unambiguous confirmation of the spin nature of R NL , we also study the Hanle effect in our devices. Only the SHE should result in an oscillatory signal due to the precession of spins in an in-plane field B || (ref. 31 ). Figure 2d compares the R NL versus B || for a CVDG sample with that of a representative EPG sample (inset). The sample dimensions in both cases are identical and their charge mobilities comparable. As expected, only the CVDG samples show a non-monotonic oscillatory dependence of the non-local signal, within the diffusive regime, and can be fitted with [31] (where ω B =Γ B || is the Larmor frequency with Γ the gyromagnetic ratio for electron and B || is the applied in-plane magnetic field). The fitting gives a λ s of 2 μm and a spin Hall angle γ of ~0.17. Control experiments The non-local length, width and Hanle precession measurements all confirm the spin origin of the R NL and give comparable values for both λ s and γ . These spin parameters are consistent with the values obtained from both independent conventional non-local spin-valve measurements (see Supplementary Fig. 3 ) [37] and spin pumping measurements published elsewhere [38] . (It is noteworthy that the distinct configurations of the spin Hall and spin-valve experiments result in spin precession R NL curves with very different magnetic field scales (see Supplementary Figs 6 and 7 and Supplementary Note 5 for details).) Furthermore, since we do not observe SHE in EPG, the origin of the SHE in CVDG must have an extrinsic origin. In principle, it can be due to a wide range of CVD-specific defects such as wrinkles, grain boundaries, ripples, vacancies, organic residues coming from the Cu etching solution or the residual Cu adatoms [21] . We can immediately rule out structural defects as the main contributor to the observed R NL since Raman mapping shows negligible D-peak for the entire device and is similar to the Raman mapping of our EPG devices (see Supplementary Fig. 1 ). We further rule out organic residues as the dominant source by immersing identically prepared exfoliated graphene samples in the same Cu etching solution (ammonium per sulphate). In such devices, the measured R NL are much smaller than in CVDG and remain comparable to the expected Ohmic contribution (see Supplementary Figs 8 and 9 and Supplementary Note 6 ). This suggests that residual Cu adatoms are the main cause for the large increase of R NL. While the density and cluster size of Cu adatoms strongly depends on the details of the etching and transfer process for CVD graphene, they are generally speaking unavoidable. This has recently also been directly confirmed by transmission electron microscopy measurements [21] . Indeed, detailed XPS and EDX measurements of our own CVDG samples confirm (see Fig. 1b ) the presence of Cu. For the samples discussed here, atomic force microscopy (AFM) measurements show Cu adatom clustering with an average size of ~20 nm in radius and particle density of 0.6 × 10 10 cm −2 (see Supplementary Fig. 10 and Supplementary Table 1 ). Note also, that here and unlike in ref. 5 , a comparison of the Raman G-peak position in CVDG with that in EPG rules out bond-angle deformation as a potential cause for the SOC enhancement [39] : while in hydrogenated graphene the Raman G-peak shows a shift of ~10 cm −1 in wavenumber [39] , a negligible G-peak shift in our CVDG demonstrates the physisorbed nature of the Cu adatoms (see Supplementary Fig. 11 and Supplementary Note 7 ). All this strongly suggests proximity-induced enhancement of the SOC. But to unambiguously establish that physisorbed Cu adatoms are the dominant cause for the observed SHE, we exfoliate graphene onto a Cu foil and repeat the same etching and transfer process used for CVD graphene (see Methods for sample preparation details). Lastly, we also perform similar measurements on EPG samples decorated with Ag and Au by both solution process and thermal evaporation (see Methods for sample preparation details). 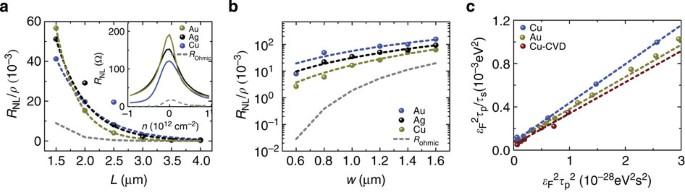Figure 3: Non-local measurements on exfoliated graphene with metallic nanoparticles. (a,b) Length and width dependence of the non-local signal for exfoliated graphene decorated with Cu, Ag and Au adatoms. The grey dotted line shows the measured non-local signal (which is equal to the Ohmic contribution) for a pristine graphene sample. (Inset:RNLversusn) (c) the Fermi-energy dependence of the spin relaxation time for various adatoms. Figure 3 summarizes the length, width and Fermi-energy dependence of the non-local signal for all three types of metal decoration. In all such samples, we do observe a R NL comparable to the one observed for CVDG samples. The fits give comparable spin relaxation lengths and spin Hall angle (see Table 1 ). In contrast to EPG dipped in etching solution only, EPG samples that have been intentionally decorated with metallic adatoms show again an oscillatory behaviour when an in-plane magnetic field is applied (see Fig. 4a,b ). This unambiguously confirms the spin origin of the non-local signal also in these samples. Figure 3: Non-local measurements on exfoliated graphene with metallic nanoparticles. ( a , b ) Length and width dependence of the non-local signal for exfoliated graphene decorated with Cu, Ag and Au adatoms. The grey dotted line shows the measured non-local signal (which is equal to the Ohmic contribution) for a pristine graphene sample. (Inset: R NL versus n ) ( c ) the Fermi-energy dependence of the spin relaxation time for various adatoms. Full size image Table 1 Graphene decorated with metallic adatoms. 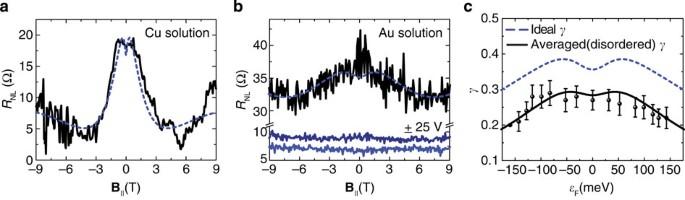Figure 4: Magnetic field dependence. In-plane magnetic field precession measurements for graphene with Cu and Au adatoms (a) Exfoliated graphene with Cu adatoms (b) exfoliated graphene with Au adatoms. Far away from the charge neutrality point the amplitude of the oscillatory behaviour of the spin signal diminishes (seeSupplementary Figs 6 and 7for additional data). The blue dashed lines are fit to the experimental data using equation (6). TheL/w=3 for all the samples with comparable mobility ~10,000 cm2V−1s−1. (c) The Fermi-energy dependence of the spin Hall coefficient,γ, for Cu-CVD graphene extracted from the length dependence data and theoretically calculated Fermi-energy dependence ofγin the resonant scattering regime taking into account Cu adatoms and other impurities limiting charge transport (seeSupplementary Note 8for the details of the calculations). The data points are from fitting the length dependence at the specified Fermi-energy and the error bar corresponds to the s.e. forγobtained from the fitting. Full size table Figure 4: Magnetic field dependence. In-plane magnetic field precession measurements for graphene with Cu and Au adatoms ( a ) Exfoliated graphene with Cu adatoms ( b ) exfoliated graphene with Au adatoms. Far away from the charge neutrality point the amplitude of the oscillatory behaviour of the spin signal diminishes (see Supplementary Figs 6 and 7 for additional data). The blue dashed lines are fit to the experimental data using equation (6). The L/w =3 for all the samples with comparable mobility ~10,000 cm 2 V −1 s −1 . ( c ) The Fermi-energy dependence of the spin Hall coefficient, γ , for Cu-CVD graphene extracted from the length dependence data and theoretically calculated Fermi-energy dependence of γ in the resonant scattering regime taking into account Cu adatoms and other impurities limiting charge transport (see Supplementary Note 8 for the details of the calculations). The data points are from fitting the length dependence at the specified Fermi-energy and the error bar corresponds to the s.e. for γ obtained from the fitting. Full size image We are now ready to estimate the SOC (Δ) in CVDG and EPG decorated with metallic adatoms. In graphene, both Elliott–Yafet (EY) and D’yakonov–Perel (DP) spin relaxation mechanisms are present. The total spin scattering rate is the sum of the individual scattering rates, that is, , where gives the EY spin relaxation due to intrinsic SOC and gives the DP spin relaxation. (Here, a =2 ( a =1) for intrinsic-like (Rashba-like) SOC [40] .) The interpretation of the experimental spin Hall angle using a semi-classical model for the adatom clusters (see Supplementary Note 8 ) suggests that the predominant contribution to the SOC enhancement comes from intrinsic-like spin–orbit interaction (see Supplementary Note 8 ), and thus we set a =2 hereafter. Following ref. 41 , we plot versus . From the slope and the y intercept, the SOC strength contribution from both the EY and DP spin relaxation can be estimated ( Fig. 3c ). Our data suggest that for all metallic adatoms, the contribution from EY spin scattering dominates over DP. The estimated Δ is only weakly dependent on the atomic number Z and falls in the range of 15±2.3 meV for CVDG and EPG decorated with Cu adatoms and 18±2 meV for EPG decorated with Au adatoms. Note that similar to metallic thin films such a weak dependence of Z is expected [42] . Finally, we discuss how metallic adatoms lead to a robust SHE with such a large γ. A large γ in pure metals such as Pt (0.01−0.1) has been ascribed to resonant scattering on impurity states split by the spin–orbit interaction [25] , [43] . The importance of such resonant scatterers in graphene is also well established [8] , [44] . The extrinsic SHE originates in asymmetric scattering in the presence of SOC: charge carriers of opposite spins are deflected in opposite directions transverse to the applied electric field. Two extrinsic mechanisms produce SHE: skew scattering (SS) and quantum-side jump (QSJ) [45] . The former arises from asymmetry of cross sections in up/down spin channels. On the other hand, QSJ produces anomalous spin currents via spin-dependent shift (side jump) of wave packets in materials endowed with momentum–space Berry curvature. Although the latter is negligible in pristine graphene (due to very weak SOC), non-trivial Berry phase-related effects emerge in adatom-doped graphene via proximity-induced effect. In the SS (QSJ) scenario, the magnitude of induced spin currents is proportional to (ref. 45 ), where n SO denotes the density of SOC active adatoms. Since all samples measured are relatively clean (that is, small n SO ) we expect SS to be critical. To identify the SHE-driving mechanism, we carried out realistic transport calculations taking into account adatoms originating the observed SOC enhancement and uncontrolled sources of disorder diminishing the delivered spin Hall angle (see Supplementary Figs 12 and 13 and Supplementary Note 8 for details). Our results confirm the dominance of SS mechanism in the experiments and show that the γ for CVDG in and around the neutrality point (±1 × 10 12 cm −2 ) remains almost a constant, due to the wide distribution of adatom cluster sizes (see Fig. 4c ). This is significant in applications for it allows the generation of robust spin currents irrespective of the initial doping level in graphene. The combination of enhanced SOC and the resonant character of large Cu clusters ( R ~20 nm) make the SS mechanism extremely efficient in the production of spin currents with giant γ in the range 0.1–0.3. With respect to the absence of a strong Z dependence, it is important to note that a large SOC at the impurity site is not the only criteria that can give rise to a large SHE. A strong perturbation of the potential at the impurity site can become equally important [42] . Indeed, in both CVD and EPG, the perturbation of the potential–due to the presence of metallic adatom clusters-is large and thus is likely the dominant mechanism. In conclusion, we have shown that the Cu-CVD graphene has a SOC three orders of magnitude larger than that of pristine exfoliated graphene samples. The enhancement in the SOC in Cu-CVD graphene is due to the presence of residual Cu adatoms introduced during the growth and transfer process. We confirm this by introducing Cu adatoms to exfoliated graphene samples and extract a SOC value comparable to the one in Cu-CVD graphene ~15 meV. In addition to Cu, we also show that adatoms like Au and Ag can also be used to induce such enhancement of SOC in pristine graphene. An enhancement of graphene’s SOC is key to achieving a robust 2D TI state in graphene. Crucially, SEM/AFM shows that in our decorations adatoms form sizeable clusters (~20 nm size), and thus severe issues associated with inter-valley scattering from isolated adatoms—such as the suppression of SHE [13] and topologically protected edge states [6] , [7] —can be largely avoided in the present scheme. Also, the observation of a robust SHE with exceptionally large γ ~0.2 at room temperature is a first but important step towards introducing graphene for spin-based concepts such as spin transfer torque based magnetic memory and spin logic applications [3] . Since the effect is equally strong with commonly used non-magnetic metals such as Cu, these applications would be also compatible with existing CMOS technology. Sample preparations Cu-CVD graphene : The growth of CVD graphene on Cu foil and the subsequent etching of Cu in ammonium per sulphate (7 g dissolved in 1 l of deionized (DI) water) and transfer onto a Si/SiO 2 substrate are performed following ref. 17 . The transferred samples are annealed in Argon/Hydrogen (90:10) environment at 320 °C for 5 h to remove any organic contaminants. Supplementary Figure 10 shows the AFM image of a graphene sample decorated with Cu nanoparticles with average particle diameter of ~40 nm and is in good agreement with the recent transmission electron microscopy results [21] . Exfoliated graphene devices with Cu adatom : The graphene samples are first exfoliated onto a SiO2 substrate with Au markers. Using the standard transfer technique for graphene/boron nitride hetero-structures [46] , the exfoliated graphene samples together with the Au markers are peeled off with a polymer layer and then transferred onto a Cu foil. The transferred samples are first baked at 120 °C in a hot plate for better adhesion. The sample on Cu foil is then placed in the Cu etchant (ammonium per sulphate, 7 g dissolved in 1 l of DI water). The etching process, which is exactly the same as the process performed for CVD graphene [17] , introduces Cu particles on graphene. A second way to introduce the Cu adatoms is to dissolve the Cu foil in the Cu etchant (ammonium per sulphate). This is followed by immersion of the final graphene spin Hall device on SiO 2 into the solution containing dissolved Cu. Exfoliated graphene devices with Au/Ag adatoms : The Au and Ag adatoms are introduced onto the graphene sample by drop casting commercially available Au/Ag colloidal solutions. The Au and Ag nanoparticles are of an average size of ~30 nm. For the experiments shown in this paper, we have used the colloidal solutions bought from BBI solutions (Product code: CIKITDIAG (for Au) and ArraySC40 (for Ag)). These solutions are diluted with DI water to get different concentrations of the nanoparticles, that is, 10 10 particles per ml to 10 7 particles per ml. For the data shown in the main text, the nanoparticle concentration is 10 8 particles per ml. The Au particles are also introduced by thermal deposition. Here, the deposition is performed using the lowest deposition rate of 0.01 Å s −1 and by opening the substrate shutter for a few seconds. This allows deposition of Au nanoparticles on graphene with an average size of ~25 nm. Supplementary Figure 10 shows the AFM image for a graphene spin Hall device with Au adatoms and Supplementary Table 1 shows the average diameter and particle distribution of various adatoms. Device fabrication The Hall bar devices are fabricated by standard e-beam lithography technique using a FEI Nova nanoSEM 230. Two steps of e-beam lithography using poly (methyl methacrylate) (PMMA Grade 950 A5 obtained from MICROCHEM) as the e-beam resist are performed for patterning the Hall bar on the graphene samples and for the introduction of Cr (~3 nm)/Au (~35 nm) contacts for transport measurements. How to cite this article: Balakrishnan, J. et al. Giant spin Hall effect in graphene grown by chemical vapour deposition. Nat. Commun. 5:4748 doi: 10.1038/ncomms5748 (2014).